PARP13 regulates cellular mRNA post-transcriptionally and functions as a pro-apoptotic factor by destabilizing TRAILR4 transcript Poly(ADP-ribose) polymerase-13 (PARP13/ZAP/ZC3HAV1) is an antiviral factor, active against specific RNA viruses such as murine leukaemia virus, Sindbis virus and human immunodeficiency virus. During infection, PARP13 binds viral RNA via its four CCCH-type zinc-finger domains and targets it for degradation by recruiting cellular messenger RNA (mRNA) decay factors such as the exosome complex and XRN1. Here we show that PARP13 binds to and regulates cellular mRNAs in the absence of viral infection. Knockdown of PARP13 results in the misregulation of hundreds of transcripts. Among the most upregulated transcripts is TRAILR4 that encodes a decoy receptor for TRAIL—a pro-apoptotic cytokine that is a promising target for the therapeutic inhibition of cancers. PARP13 destabilizes TRAILR4 mRNA post-transcriptionally in an exosome-dependent manner by binding to a region in its 3′ untranslated region. As a consequence, PARP13 represses TRAILR4 expression and increases cell sensitivity to TRAIL-mediated apoptosis, acting as a key regulator of the cellular response to TRAIL. Poly(ADP-ribose) polymerase-13 (PARP13), also known as zinc-finger antiviral protein, ARTD13 and ZC3HAV1, is a member of the PARP family of proteins—enzymes that modify target proteins with adenosine diphosphate (ADP)-ribose using nicotinamide adenine dinucleotide (NAD + ) as substrate [1] . Two PARP13 isoforms are expressed constitutively in human cells: PARP13.1 is targeted to membranes by a C-terminal CaaX motif, whereas PARP13.2 is cytoplasmic [1] , [2] . Both proteins are unable to generate ADP-ribose—PARP13.1 contains a PARP domain lacking key amino-acid residues required for PARP activity, whereas the entire PARP domain is absent in PARP13.2 (ref. 1 ). Both isoforms of PARP13 contain four N-terminal RNA-binding CCCH-type zinc finger—domains found in proteins that function in the regulation of RNA stability and splicing such as tristetraprolin and muscleblind-like (MBNL1), respectively [3] , [4] , [5] , [6] . PARP13 was originally identified in a screen for antiviral factors [3] . It binds RNAs of viral origin during infection and targets them for degradation via the cellular messenger RNA (mRNA) decay machinery [7] , [8] , [9] . Several RNA viruses, including murine leukaemia virus, Sindbis virus, human immunodeficiency virus and Epstein–Barr virus as well as the RNA intermediate of the hepatitis B DNA virus have been shown to be targets of PARP13 (refs 3 , 7 , 8 , 10 , 11 , 12 ). How viral RNA is detected by PARP13 is currently not known, and although binding to PARP13 is a requirement for viral RNA degradation, no motifs or structural features common to the known targets have been identified [13] . Structure analysis of the PARP13 RNA-binding domain suggests that PARP13 binds looped RNA, therefore target recognition could involve structural features rather than linear sequence motifs [6] . PARP13 binds to multiple components of the cellular 3′–5′ mRNA decay machinery including polyA-specific ribonuclease, and subunits of the exosome exonuclease complex, RRP46/EXOSC5 and RRP42/EXOSC7 (refs 8 , 9 ). Recruitment of these decay factors results in the 3′–5′ cleavage of viral RNAs bound to PARP13. Although 5′–3′ RNA decay has also been shown to play a role in PARP13-mediated viral degradation, proteins involved in this process including the decapping factors DCP1 and DCP2 and the 5′–3′ exonuclease XRN1, do not bind to PARP13 directly and are instead recruited by other PARP13-binding partners such as DDX17 (ref. 8 ). Whether or not PARP13 binds to and modulates cellular RNAs either in the absence or presence of viral infection is unknown. However, several indications point towards a role for PARP13 in cellular RNA regulation: (1) both PARP13 isoforms are expressed at high levels in cells, however, only PARP13.2 expression is upregulated during viral infection suggesting that PARP13.1 has functions unrelated to the antiviral response [1] , [14] ; (2) even in the absence of viral infection, PARP13 localizes to RNA-rich stress granules—non-membranous ribonucleoprotein structures that form during cellular stress to sequester mRNAs and inhibit their translation [15] ; (3) PARP13 regulates the microRNA (miRNA) pathway by targeting Argonaute proteins for ADP-ribosylation and this regulation occurs both in the absence and in the presence of viral infection [15] , [16] . This suggests that PARP13 targeting of RNA to cellular decay pathways could also occur in the absence of viral infection, and that PARP13 could therefore function as a general regulator of cellular mRNA. Here we show that PARP13 binds to and regulates cellular RNA in the absence of viral infection, and that its depletion results in significant misregulation of the transcriptome with an enrichment in signal peptide-containing transcripts and immune response genes. From the list of PARP13-dependent differentially expressed genes we focused this study on understanding how PARP13 regulates TRAILR4—a member of a family of transmembrane receptors composed of TRAILR1-4 (refs 17 , 18 ) that bind to TRAIL, a pro-apoptotic tumour necrosis factor-family cytokine. We show that PARP13 destabilizes TRAILR4 mRNA post-transcriptionally but has no effect on the levels of other TRAIL receptors. It binds to a specific fragment in the 3′ untranslated region (3′UTR) of TRAILR4 mRNA, and leads to its degradation via the RNA exosome complex. Primary cells are TRAIL resistant; however, many transformed cells become sensitive to TRAIL-induced apoptosis, making it an attractive target for the therapeutic treatment of cancers [17] . TRAIL binding to TRAILR1 and TRAILR2 triggers the assembly of the death-inducing signalling complex (DISC) [19] , [20] leading to the recruitment and activation of caspase-8 and the induction of the extrinsic apoptotic pathway [19] , [20] . In contrast, TRAILR3 and TRAILR4 act as prosurvival decoy receptors that bind TRAIL but cannot assemble functional DISCs and therefore cannot signal apoptosis [21] , [22] . The relative expression of each receptor varies in different cancers and tissue types and is thought to be important for the overall cellular response to TRAIL [23] . Accordingly, high levels of these decoy receptors can prevent TRAIL-induced cell death and likely contribute to acquired TRAIL resistance in cancer cells [24] . By repressing TRAILR4 expression PARP13 acts a key regulator of the cellular response to TRAIL, and depletion of PARP13 results in TRAILR4 protein accumulation and TRAIL resistance in multiple cell lines. PARP13 binds to cellular RNA To determine whether PARP13 binds to cellular RNA, we performed crosslinking immunopreciptation (CLIP) in HeLa cells using affinity purified PARP13 antibody. A strong signal from bound, crosslinked RNA that collapsed to two major bands at high RNase concentrations was identified ( Fig. 1a ). The collapsed signal migrated at the molecular weight of PARP13.1 and 13.2, and was PARP13 specific since it was not detected in similar purifications performed in PARP13 −/− HeLa cell lines generated using zinc-finger nucleases ( Fig. 1a ; Supplementary Fig. 1 ). Since PARP13.1 and PARP13.2 are constitutively expressed in HeLa cells, we compared the binding of cellular RNA with each isoform using N-terminal streptavidin-binding protein (SBP) fusions. SBP-PARP13.1 and SBP-PARP13.2 bound similar amounts of RNA, and the signal for both was RNAse sensitive confirming the attached molecules as RNA ( Fig. 1b,c ). For both the endogenous PARP13 and the SBP precipitations no signal was identified when ultraviolet crosslinking was omitted demonstrating the specificity of the reactions ( Fig. 1d ). To further confirm that binding of RNA to PARP13 is specific and requires the CCCH zinc-fingers, we generated deletions of these domains from PARP13.1 and PARP13.2 and performed CLIP (PARP13.1 ΔZnF and PARP13.2 ΔZnF ) ( Fig. 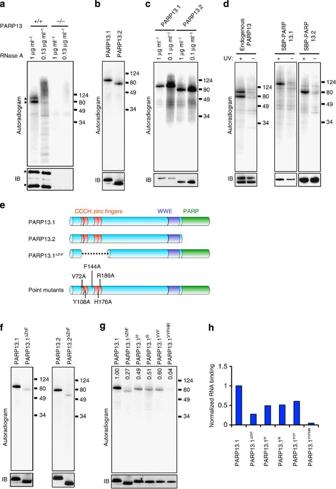Figure 1: PARP13 binds cellular RNA. (a) Autoradiogram of PARP13 CLIP reactions performed using wild-type (+/+) or PARP13-null (−/−) cells treated with 1 μg ml−1or 0.13 μg ml−1RNaseA. Triangle indicates molecular weight (MW) of PARP13.1, circle indicates MW of PARP13.2. PARP13 immunoblot (IB) shown below. (b) Autoradiogram of CLIP reactions from SBP-PARP13.1 and PARP13.2 expressed and purified in wild-type cells treated with 1 μg ml−1RNaseA. PARP13 immunoblots shown below. (c) Autoradiogram of SBP-PARP13.1 and SBP-PARP13.2 CLIP reactions treated with 1 or 0.1 μg ml−1RNase A. PARP13 immunoblots are shown below. (d) CLIP autoradiograms of endogenous PARP13, SBP-PARP13.1 and SBP-PARP13.2 treated with 1 μg ml−1RNase A with or without ultraviolet crosslinking (254 nm, 200 mJ). PARP13 immunoblots shown below. (e) Diagram of PARP13 isoforms and mutants. (f) CLIP autoradiograms of SBP-PARP13.1, PARP13.1ΔZnF, PARP13.2 and PARP13.2ΔZnFprecipitations treated with 1 μg ml−1RNase A. PARP13 immunoblot shown below. (g) Autoradiogram of wild-type and mutant PARP13.1 CLIP reactions. PARP13 immunoblot shown below (IB). Numerical values of32P signal normalized to protein levels shown above; PARP13.1 RNA-binding levels set to 1. (h) Graph of32P signals normalized to PARP13.1 protein levels for CLIP analysis shown ing. 1e,f , Table 1 ). Deletion of these domains resulted in marked reduction of the signal. Figure 1: PARP13 binds cellular RNA. ( a ) Autoradiogram of PARP13 CLIP reactions performed using wild-type (+/+) or PARP13-null (−/−) cells treated with 1 μg ml −1 or 0.13 μg ml −1 RNaseA. Triangle indicates molecular weight (MW) of PARP13.1, circle indicates MW of PARP13.2. PARP13 immunoblot (IB) shown below. ( b ) Autoradiogram of CLIP reactions from SBP-PARP13.1 and PARP13.2 expressed and purified in wild-type cells treated with 1 μg ml −1 RNaseA. PARP13 immunoblots shown below. ( c ) Autoradiogram of SBP-PARP13.1 and SBP-PARP13.2 CLIP reactions treated with 1 or 0.1 μg ml −1 RNase A. PARP13 immunoblots are shown below. ( d ) CLIP autoradiograms of endogenous PARP13, SBP-PARP13.1 and SBP-PARP13.2 treated with 1 μg ml −1 RNase A with or without ultraviolet crosslinking (254 nm, 200 mJ). PARP13 immunoblots shown below. ( e ) Diagram of PARP13 isoforms and mutants. ( f ) CLIP autoradiograms of SBP-PARP13.1, PARP13.1 ΔZnF , PARP13.2 and PARP13.2 ΔZnF precipitations treated with 1 μg ml −1 RNase A. PARP13 immunoblot shown below. ( g ) Autoradiogram of wild-type and mutant PARP13.1 CLIP reactions. PARP13 immunoblot shown below (IB). Numerical values of 32 P signal normalized to protein levels shown above; PARP13.1 RNA-binding levels set to 1. ( h ) Graph of 32 P signals normalized to PARP13.1 protein levels for CLIP analysis shown in g . Full size image Table 1 PARP13 RNA-binding mutants used in this manuscript. Full size table Structural analysis of the PARP13 RNA-binding domain containing four CCCH zinc-fingers identified key amino-acid residues for viral RNA binding [6] . Two cavities, defined by V72, Y108, F144 (cavity 1) and H176, R189 (cavity 2) are thought to be important for RNA binding. We mutated each residue of cavity 1, multiple residues in cavity 2 and all five residues found in both cavities to alanine in SBP-PARP13.1 and assayed the mutants for RNA binding using CLIP ( Fig. 1e,g , Table 1 ). Mutation of all five residues to generate PARP13.1 VYFHR reduced RNA binding to negligible levels and mutation of all three cavity-1 residues resulted in a similar decrease in RNA binding as individual mutations of each cavity-2 residue ( Fig. 1g,h ). It is possible that the reduction in RNA binding in the mutants was a result of aggregation or mislocailzation of the mutant proteins. To test this, we compared the localization of PARP13.1 ΔZnF and PARP13.1 VYFHR with that of wild-type protein in HeLa cells. Both mutants exhibited localization patterns similar to PARP13.1 ( Fig. 2 ). We also examined localization of the mutant proteins to stress granules. We previously showed that PARP13 is highly enriched in stress granules, structures that are assembled during cytoplasmic stress and contain high concentrations of cellular mRNA [15] . PARP13.1 properly localized to stress granules upon sodium arsenite treatment, however, both PARP13.1 ΔZnF and PARP13.1 VYFHR failed to localize to these structures [15] , [25] ( Fig. 2 ; Supplementary Fig. 2 ). This defective targeting was even more striking for PARP13.2 ΔZnF and PARP13.2 VYFHR ( Fig. 2 ; Supplementary Fig. 2 ). These results confirm that the mutants are defective in binding RNA and that this defect affects cellular function. They further suggest that binding to cellular RNA is critical for PARP13 localization to stress granules. 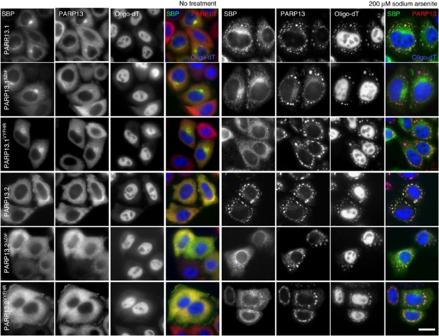Figure 2: Localization of PARP13.1, PARP13.2 and RNA-binding mutants. Immunofluorescence showing co-staining of exogenously expressed PARP13.1, PARP13.1ΔZnF, PARP13.1VYFHR, PARP13.2, PARP13.2ΔZnFor PARP13.2VYFHRin non-stressed (no treatment) and stressed (200 μM sodium arsenite) cells. Scale Bar, 20 μm. Figure 2: Localization of PARP13.1, PARP13.2 and RNA-binding mutants. Immunofluorescence showing co-staining of exogenously expressed PARP13.1, PARP13.1 ΔZnF , PARP13.1 VYFHR , PARP13.2, PARP13.2 ΔZnF or PARP13.2 VYFHR in non-stressed (no treatment) and stressed (200 μM sodium arsenite) cells. Scale Bar, 20 μm. Full size image PARP13 regulates the transcriptome To determine whether PARP13 regulates cellular RNA, we analysed the transcriptome in the absence of PARP13. We used Agilent microarrays to compare the relative abundance of transcripts in HeLa cells transfected with control short interfering RNA (siRNA) to cells transfected with PARP13-specific siRNA ( Fig. 3a ; Supplementary Data 1 ). Depletion of PARP13 resulted in significant misregulation of the transcriptome with 1,841 out of a total of 36,338 transcripts analysed showing >0.5 Log2 fold change (Log2FC) relative to control knockdowns (1,065 upregulated and 776 downregulated transcripts). Of these, 85 transcripts exhibited Log2FC>1 relative to control siRNAs (66 upregulated and 19 downregulated). In total, 73 transcripts passed a significance threshold of P <0.05 (moderated t -statistic with the Benjamini–Hochberg adjustment) ( Table 2 ). 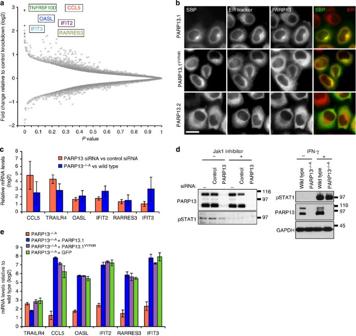Figure 3: PARP13-depletion results in misregulation of the transcriptome. (a) Volcano plot showing transcriptome-wide Log2 fold changes in mRNA expression in PARP13 knockdowns relative to control knockdowns obtained via Agilent array analysis of total mRNA (n=2 independent experiments). Six of the top 10 upregulated transcripts are labelled. The remaining mRNA data shown in the figure were obtained using qRT-PCR. (b) Immunofluorescence of cells expressing SBP-PARP13.1, SBP-PARP13.1VYFHRor SBP-PARP13.2, stained with anti-PARP13 and anti-SBP antibodies, and ER Tracker Red. In merge SBP signal is in green, ER Tracker signal is in red, PARP13 signal is not shown. Scale bar, 20 μm. (c) Confirmation of CCL5, TRAILR4, OASL, IFIT2, RARRES3 and IFIT3 upregulation in PARP13 knockdown relative to control knockdown and in PARP13−/−AHeLa cells relative to wild-type cells (n=3 independent experiments, bars represent s.d.). (d) Left, immunoblots of PARP13 and pSTAT1 in untransfected cells, or cells transfected with control or PARP13-specific siRNA, untreated or treated with 5 μM Jak1 inhibitor; right, immunoblots of PARP13 and pSTAT1 in wild-type and PARP13−/−HeLa cells untreated or treated with 100 units ml−1interferon (IFN)γ. GAPDH shown as loading control. (e) mRNA levels of TRAILR4, CCL5, OASL, IFIT2, RARRES3 and IFIT3 in untransfected PARP13−/−cells and PARP13−/−cells expressing PARP13.1, PARP13.1VYFHRor GFP (DNA transfection control) relative to HeLa cells (n=3 independent experiments, bars represent s.d.). Figure 3: PARP13-depletion results in misregulation of the transcriptome. ( a ) Volcano plot showing transcriptome-wide Log2 fold changes in mRNA expression in PARP13 knockdowns relative to control knockdowns obtained via Agilent array analysis of total mRNA ( n =2 independent experiments). Six of the top 10 upregulated transcripts are labelled. The remaining mRNA data shown in the figure were obtained using qRT-PCR. ( b ) Immunofluorescence of cells expressing SBP-PARP13.1, SBP-PARP13.1 VYFHR or SBP-PARP13.2, stained with anti-PARP13 and anti-SBP antibodies, and ER Tracker Red. In merge SBP signal is in green, ER Tracker signal is in red, PARP13 signal is not shown. Scale bar, 20 μm. ( c ) Confirmation of CCL5, TRAILR4, OASL, IFIT2, RARRES3 and IFIT3 upregulation in PARP13 knockdown relative to control knockdown and in PARP13 −/−A HeLa cells relative to wild-type cells ( n =3 independent experiments, bars represent s.d.). ( d ) Left, immunoblots of PARP13 and pSTAT1 in untransfected cells, or cells transfected with control or PARP13-specific siRNA, untreated or treated with 5 μM Jak1 inhibitor; right, immunoblots of PARP13 and pSTAT1 in wild-type and PARP13 −/− HeLa cells untreated or treated with 100 units ml −1 interferon (IFN)γ. GAPDH shown as loading control. ( e ) mRNA levels of TRAILR4, CCL5, OASL, IFIT2, RARRES3 and IFIT3 in untransfected PARP13 −/− cells and PARP13 −/− cells expressing PARP13.1, PARP13.1 VYFHR or GFP (DNA transfection control) relative to HeLa cells ( n =3 independent experiments, bars represent s.d.). Full size image Table 2 Number of differentially expressed transcripts upon PARP13 depletion. Full size table The 50 upregulated transcripts with a P value <0.05 showed enrichment for genes containing a signal peptide required for targeting of mRNA for translation at the endoplasmic reticulum (ER) (analysed with the Database for Annotation, Visualization and Integrated Discovery [26] , Enrichment Score 3.4, P value <0.0001; Supplementary Data 2 ), suggesting that PARP13 could regulate transcripts at the ER. The membranous perinuclear localization we observed for PARP13.1 ( Fig. 2 ) and the previously reported membrane targeting of this protein [2] suggested a potential enrichment at the ER. We therefore costained exogenously expressed PARP13 isoforms with the ER marker ER Tracker, and observed colocalization with PARP13.1 but not PARP13.2. This localization is independent of RNA binding since PARP13.1 VYFHR localized very similarly to the wild-type protein ( Fig. 3b ). Targeting of PARP13 to the ER may therefore be one mechanism of regulating its function and its RNA target specificity. Gene set enrichment analysis [27] of the same genes identified enrichment for members of the interferon immune response pathway ( P value <0.0001, normalized enrichment score=2.22) ( Supplementary Fig. 3 ; Supplementary Data 3 ). To verify our results, we analysed 6 of the top 10 most upregulated transcripts using quantitative real-time reverse-transcription PCR (qRT-PCR) in both PARP13 knockdowns and PARP13 −/− cells. All six transcripts were upregulated relative to controls upon PARP13 depletion ( Fig. 3c ). With the exception of TRAILR4/TNFRSF10D, each of these genes encodes an immune response gene and is a member of the interferon-stimulated genes (ISGs), activated in response to interferon signalling. The upregulation of the five ISGs appears to be specific and is not the result of a general activation of the interferon response since JAK-STAT signalling was not increased in the knockdown or knockout cells ( Fig. 3d ) and since other canonical ISGs (interferon regulatory factors (IRFs), tripartite motif containing proteins (TRIMs) and interferon induced transmembrane proteins (IFITMs)) were not upregulated in our transcriptome analysis ( Supplementary Data 1 ). Interestingly, like PARP13, the upregulated ISGs (OASL, IFIT2 and IFIT3) function in inhibition of viral replication and translation [28] , suggesting that their upregulation could be a compensatory mechanism for PARP13 depletion. To identify the direct targets of PARP13 regulation among the six highly upregulated transcripts, we compared their expression levels in PARP13 −/− cells relative to PARP13 −/− cells expressing wild-type PARP13 or PARP13 RNA-binding mutant. While both PARP13.1 and PARP13.2 are constitutively expressed in HeLa cells, PARP13.2 expression increases during viral infection in an interferon-dependent manner, whereas PARP13.1 expression does not [14] . Therefore to exclude interferon-related effects we focused our experiments on PARP13.1. Direct targets of PARP13 RNA binding and regulation would in theory decrease upon PARP13.1, but not PARP13 VYFHR , expression in PARP13 −/− cells. TRAILR4 mRNA clearly behaved in this manner with a 40% decrease in transcript levels upon PARP13.1 expression and no change upon PARP13.1 VYFHR expression ( Fig. 3e ). This analysis proved difficult for the remaining five transcripts since transient plasmid transfection induced a transcriptional upregulation of these ISGs as previously shown [29] . PARP13 represses TRAILR4 mRNA and protein expression Owing to its biological importance and the clinical interest in TRAIL, we examined the role of PARP13 in the regulation of TRAILR4 expression and how that regulation might impact TRAIL signalling and apoptosis. Upregulation of TRAILR4 mRNA in PARP13-depleted HeLa cells had a direct effect on TRAILR4 protein expression: TRAILR4 protein levels, barely detectable in wild-type HeLa cells, increased in PARP13 knockdown cells and in all three independently isolated PARP13 −/− cell lines ( Fig. 4a,b ). In addition, consistent with our results identifying TRAILR4 as a direct target of PARP13 regulation ( Fig. 3e ; Supplementary Fig. 4 ), expression of PARP13.1, but not PARP13.1 VYFHR , in PARP13 −/−A cells was sufficient to reduce TRAILR4 protein expression ( Fig. 4c ). PARP13 repression of TRAILR4 mRNA represents a general mechanism of TRAILR4 regulation in multiple human cell types. In all cell lines tested, including primary cells such as Tert immortalized retinal primary epithelial (RPE1) cells and transformed cells such as human colon HCT116, human colon adenocarcinoma SW480 and HeLa cells, TRAILR4 mRNA levels increased upon PARP13 depletion identifying suppression of TRAILR4 expression as an important physiological function of PARP13 ( Fig. 4d ). Under physiological conditions, the primary isoform of PARP13 that regulates TRAILR4 is PARP13.1 since specific knockdown of PARP13.1 in HeLa cells increased TRAILR4 mRNA to levels similar to those obtained upon total PARP13 depletion ( Fig. 4e ). 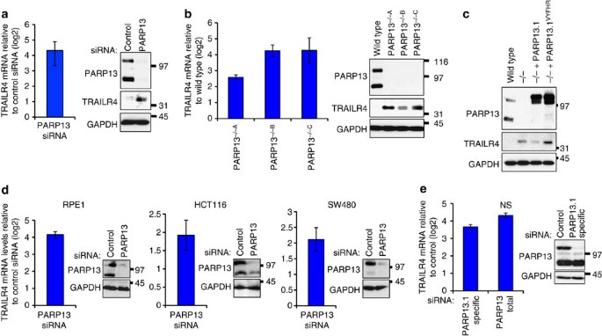Figure 4: PARP13 repression of TRAILR4 mRNA and protein levels is dependent on its RNA binding. (a) TRAILR4 mRNA and protein levels in PARP13 knockdown relative to control. GAPDH shown as a loading control.n=3 independent experiments, error bars show s.d. (b) TRAILR4 mRNA and protein levels in PARP13−/−cell lines relative to wild-type cells. GAPDH shown as a loading control.n=3 independent experiments, error bars show s.d. (c) TRAILR4 protein levels in wild-type, PARP13−/−Aand PARP13−/−Acells expressing PARP13.1 or PARP13.1VYFHR. GAPDH shown as a loading control. (d) TRAILR4 mRNA levels (Log2FC) in PARP13 knockdown relative to control knockdown in RPE1, SW480 and HCT116 cells (averages ofn=3 parallel reactions (RPE1) orn=3 independent experiments (SW480 and HCT116) shown, error bars show s.d.). Immunoblots show PARP13 knockdown; GAPDH shown as a normalizing control. (e) TRAILR4 mRNA levels in cells treated with PARP13.1-specific and total PARP13-specific siRNAs relative to control siRNAs (averages ofn=3 independent experiments shown, error bars show s.d.,P>0.05 (NS, not significant), two-sidedt-test comparing the two knockdowns). Immunoblots show PARP13.1 depletion upon knockdown with PARP13.1-specific siRNA. GAPDH shown as a loading control. Figure 4: PARP13 repression of TRAILR4 mRNA and protein levels is dependent on its RNA binding. ( a ) TRAILR4 mRNA and protein levels in PARP13 knockdown relative to control. GAPDH shown as a loading control. n =3 independent experiments, error bars show s.d. ( b ) TRAILR4 mRNA and protein levels in PARP13 −/− cell lines relative to wild-type cells. GAPDH shown as a loading control. n =3 independent experiments, error bars show s.d. ( c ) TRAILR4 protein levels in wild-type, PARP13 −/−A and PARP13 −/−A cells expressing PARP13.1 or PARP13.1 VYFHR . GAPDH shown as a loading control. ( d ) TRAILR4 mRNA levels (Log2FC) in PARP13 knockdown relative to control knockdown in RPE1, SW480 and HCT116 cells (averages of n =3 parallel reactions (RPE1) or n =3 independent experiments (SW480 and HCT116) shown, error bars show s.d.). Immunoblots show PARP13 knockdown; GAPDH shown as a normalizing control. ( e ) TRAILR4 mRNA levels in cells treated with PARP13.1-specific and total PARP13-specific siRNAs relative to control siRNAs (averages of n =3 independent experiments shown, error bars show s.d., P >0.05 (NS, not significant), two-sided t -test comparing the two knockdowns). Immunoblots show PARP13.1 depletion upon knockdown with PARP13.1-specific siRNA. GAPDH shown as a loading control. Full size image PARP13 inhibits TRAILR4 post-transcriptionally via its 3′UTR The PARP13.1 and PARP13.1 VYFHR rescue assays performed in PARP13 −/− cells suggest that TRAILR4 regulation by PARP13 is post-transcriptional and requires RNA binding to PARP13 ( Fig. 3e ; Supplementary Fig. 4 ). Post-transcriptional regulation was confirmed by analysing the upregulated TRAILR4 transcripts via qRT-PCR with primers that overlap intron–exon boundaries to identify unspliced pre-mRNA, and primers that overlap exon–exon boundaries, to identify mature transcripts. PARP13 knockdown resulted in increased amounts of mature TRAILR4 mRNA, but had no effect on the amount of pre-mRNA, suggesting that TRAILR4 transcription is not altered upon PARP13 depletion and that regulation of TRAILR4 by PARP13 is post-transcriptional ( Fig. 5a ). Since post-transcriptional regulation of mRNA often occurs via the 3′UTR, we designed reporter constructs containing the 3′UTR of TRAILR4 or glyceraldehyde 3-phosphate dehydrogenase (GAPDH) (as negative control) fused to Renilla luciferase in the psiCHECK2 vector. This vector also encodes Firefly luciferase as a transfection control. Renilla-TRAILR4 3′UTR expression was decreased ~20% in HeLa cells relative to PARP13 −/− cells, whereas no significant difference in Renilla or Renilla-GAPDH 3′UTR expression was detected between the two cell lines ( Fig. 5b ). Together these results suggest that PARP13 destabilizes TRAILR4 post-transcriptionally via its 3′UTR. 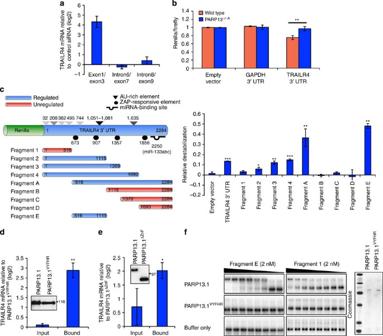Figure 5: PARP13 represses TRAILR4 mRNA post-transcriptionally by binding to a specific region in its 3′UTR. All RNA quantification performed using qRT-PCR. (a) TRAILR4 mature RNA (exon1/exon3 primer) and pre-mRNA (intron6–exon7, intron8/exon9 primers) levels in PARP13 knockdown relative to control knockdown (mean ofn=3 independent experiments, error bars show s.d.). (b) Normalized Renilla/Firefly luminescence for psiCHECK2 empty vector, psiCHECK2-expressing Renilla-GAPDH 3′UTR (GAPDH 3′UTR) and psiCHECK2-expressing Renilla-TRAILR4 3′UTR (TRAILR4 3′UTR) expressed in wild-type or PARP13−/−Acells (mean ofn=3 independent experiments, error bars represent s.d., **P<0.01, two-sidedt-test). (c) Left top, diagram of Renilla-TRAILR4 3′UTR construct identifying AU-rich elements (ARE), ZAP-responsive elements (ZRE) and miRNA-binding site for miR-133; triangle shading indicates relative length of motif—darker shades correspond to longer motifs. Specific ARE sequences and locations are shown inSupplementary Fig. 5. Left bottom, fragments used in 3′UTR destabilization assay. Blue fragments exhibited PARP13-dependent destabilization, whereas red fragments were not regulated. Right, relative PARP13-dependent destabilization for each 3′UTR fragment, represented by fraction increase of normalized Renilla luminescence in PARP13−/−Acells relative to wild-type cells (means ofn=3 independent experiments, error bars show s.d., asterisks represent significance relative to the empty vector, *P<0.05, **P<0.01 and ***P<0.001, two-sidedt-test). (d) Fold enrichment (Log2) of TRAILR4 mRNA in input and bound fraction in PARP13.1 CLIP reactions relative to PARP13.1VYFHRreactions (mean ofn=3 independent experiments, error bars show s.d., **P<0.01, two-sidedt-test). PARP13 immunoblot shows precipitated protein levels. (e) Relative Log2 levels of TRAILR4 mRNA in input and bound fractions in PARP13.1 CLIP reactions relative to PARP13.1ΔZnFreactions (averages ofn=3 independent experiments, bars show s.d., *P<0.05 relative to PARP13.1ΔZnF, two-sidedt-test). PARP13 Immunoblot of precipitated protein shown at right. (f) Electrophoretic mobility shift assays (EMSAs) of decreasing amounts of PARP13.1 and PARP13.1VYFHR(from 533 to 71 nM, in 25% interval decrease) with radiolabelled fragment E and fragment 1 (experiment was repeated three times with similar results). Right, Coomassie stain showing equal protein concentration of PARP13.1 and PARP13.1VYFHR. Figure 5: PARP13 represses TRAILR4 mRNA post-transcriptionally by binding to a specific region in its 3′UTR. All RNA quantification performed using qRT-PCR. ( a ) TRAILR4 mature RNA (exon1/exon3 primer) and pre-mRNA (intron6–exon7, intron8/exon9 primers) levels in PARP13 knockdown relative to control knockdown (mean of n =3 independent experiments, error bars show s.d.). ( b ) Normalized Renilla/Firefly luminescence for psiCHECK2 empty vector, psiCHECK2-expressing Renilla-GAPDH 3′UTR (GAPDH 3′UTR) and psiCHECK2-expressing Renilla-TRAILR4 3′UTR (TRAILR4 3′UTR) expressed in wild-type or PARP13 −/−A cells (mean of n =3 independent experiments, error bars represent s.d., ** P <0.01, two-sided t -test). ( c ) Left top, diagram of Renilla-TRAILR4 3′UTR construct identifying AU-rich elements (ARE), ZAP-responsive elements (ZRE) and miRNA-binding site for miR-133; triangle shading indicates relative length of motif—darker shades correspond to longer motifs. Specific ARE sequences and locations are shown in Supplementary Fig. 5 . Left bottom, fragments used in 3′UTR destabilization assay. Blue fragments exhibited PARP13-dependent destabilization, whereas red fragments were not regulated. Right, relative PARP13-dependent destabilization for each 3′UTR fragment, represented by fraction increase of normalized Renilla luminescence in PARP13 −/−A cells relative to wild-type cells (means of n =3 independent experiments, error bars show s.d., asterisks represent significance relative to the empty vector, * P <0.05, ** P <0.01 and *** P <0.001, two-sided t -test). ( d ) Fold enrichment (Log2) of TRAILR4 mRNA in input and bound fraction in PARP13.1 CLIP reactions relative to PARP13.1 VYFHR reactions (mean of n =3 independent experiments, error bars show s.d., ** P <0.01, two-sided t -test). PARP13 immunoblot shows precipitated protein levels. ( e ) Relative Log2 levels of TRAILR4 mRNA in input and bound fractions in PARP13.1 CLIP reactions relative to PARP13.1 ΔZnF reactions (averages of n =3 independent experiments, bars show s.d., * P <0.05 relative to PARP13.1 ΔZnF , two-sided t -test). PARP13 Immunoblot of precipitated protein shown at right. ( f ) Electrophoretic mobility shift assays (EMSAs) of decreasing amounts of PARP13.1 and PARP13.1 VYFHR (from 533 to 71 nM, in 25% interval decrease) with radiolabelled fragment E and fragment 1 (experiment was repeated three times with similar results). Right, Coomassie stain showing equal protein concentration of PARP13.1 and PARP13.1 VYFHR . Full size image Computational analysis of the TRAILR4 3′UTR identified seven putative AU-rich elements (AREs) known to destabilize RNA [30] , [31] , one conserved miRNA-binding site that is muscle specific (miR-133abc) [32] , [33] and four short and poorly characterized zinc-finger antiviral protein-responsive elements (ZREs) predicted by SELEX to mediate PARP13 recognition of RNA targets [13] ( Fig. 5c ; Supplementary Fig. 5 ). To identify the key PARP13-dependent regulatory sequences in the TRAILR4 3′UTR, we designed truncations of the TRAILR4 3′UTR and fused them to Renilla luciferase in the psiCHECK2 vector ( Fig. 5c ). Fragments were designed based on a secondary structure prediction of the TRAILR4 3′UTR to avoid disturbing high-probability RNA folds [34] ( Supplementary Fig. 6 ). The relative PARP13-dependent destabilization of each fragment was determined by subtracting expression in wild-type cells from expression in PARP13 −/− cells ( Fig. 5c ; Supplementary Fig. 7 ). This analysis identified nucleotides 516–1115 of the 3′UTR as necessary for PARP13 regulation. Fusion of nucleotides 516–1115 (fragment E) to Renilla resulted in destabilization of the construct in wild-type cells, confirming that this sequence contains the relevant signal for PARP13-dependent repression ( Fig. 5c ). This fragment includes two ZREs and two AREs, including one that contains multiple overlapping ARE sequences suggesting that PARP13 regulation of TRAILR4 mRNA might require ARE and/or ZRE recognition. Our analysis also suggests that TRAILR4 regulation is likely miRNA independent since no predicted miRNA-binding sites are found in the TRAILR4 regulatory sequence. PARP13 binds TRAILR4 mRNA To determine whether PARP13 regulation of TRAILR4 occurs via direct binding to TRAILR4 mRNA, we performed CLIP qRT-PCR in cells expressing SBP-PARP13.1, SBP-PARP13.1 VYFHR or PARP13.1 ΔZnF and electrophoretic mobility shift assays (EMSAs) using purified SBP-PARP13.1 or SBP-PARP13.1 VYFHR and 32 P-labelled fragment E or fragment 1 as control. CLIP qRT-PCR analysis identified significant enrichment of TRAILR4 mRNA in wild-type PARP13.1 precipitations relative to PARP13.1 VYFHR or PARP13.1 ΔZnF , confirming a direct and specific binding interaction between TRAILR4 mRNA and PARP13 in vivo ( Fig. 5d,e ). These results were confirmed in vitro by EMSAs where SBP-PARP13.1 bound to fragment E with high affinity (Kd=123 nM) and to fragment 1 with lower affinity (Kd=508 nM). PARP13.1 VYFHR failed to bind either fragment ( Fig. 5f ). These experiments demonstrate the specificity of TRAILR4 mRNA binding to PARP13 and show that the regulatory region of the TRAILR4 3′UTR binds directly to PARP13 with good selectivity ( Fig. 5f ). PARP13 destabilization of TRAILR4 mRNA is exosome dependent PARP13 regulates viral RNA stability via XRN1-dependent 5′–3′ decay, and exosome-dependent 3′–5′ decay [8] . PARP13 can also bind to and modulate Argonaute (Ago) activity, critical for miRNA-dependent post-transcriptional regulation of mRNA stability [15] . To determine whether TRAILR4 mRNA stability is regulated through any of these pathways, TRAILR4 mRNA levels were examined upon knockdown of Ago2, XRN1 or EXOSC5, an exosome complex component shown to bind PARP13 (ref. 9 ). Knockdown of EXOSC5, verified by qRT-PCR (antibodies were non-reactive), resulted in stabilization of TRAILR4 mRNA in HeLa cells suggesting that exosome function is necessary for regulation of TRAILR4 mRNA ( Fig. 6a,b ). In contrast, neither XRN1 knockdown in HeLa cells nor depletion of Ago2 in HEK293 cells using tetracycline-inducible Ago2 short hairpin RNA [35] resulted in obvious TRAILR4 mRNA stabilization ( Fig. 6a–c ). PARP13 depletion in the Ago2 short hairpin RNA-inducible cell lines resulted in similar levels of TRAILR4 upregulation regardless of Ago2 depletion, further suggesting that Ago2 function is not necessary for TRAILR4 regulation by PARP13 ( Fig. 6c ). 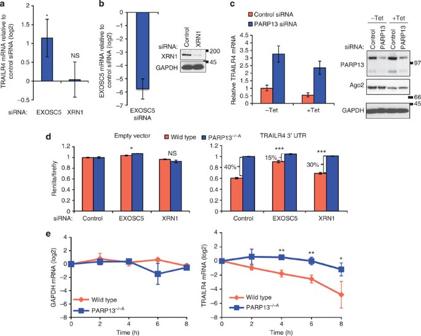Figure 6: PARP13 destabilization of TRAILR4 mRNA is exosome dependent. (a) TRAILR4 mRNA levels in EXOSC5 and XRN1 knockdowns relative to control knockdown (means ofn=3 independent experiments, bars show s.d., asterisks represent significance relative to control siRNA, *P<0.05,P>0.05 (NS, not significant), two-sidedt-test). (b) Left, EXOSC5 mRNA levels in EXOSC5 knockdown relative to control knockdown (bars show s.d.,n=3 independent experiments); right, immunoblot showing XRN1 protein levels in control and XRN1 knockdown. GAPDH is shown as a loading control. (c) Relative TRAILR4 mRNA levels in Tet-treated or untreated HEK293 cells expressing Tet-inducible Ago2 shRNA, treated with control or PARP13-specific siRNA (averages ofn=3 parallel reactions, error bars show s.d.). Immunoblots of PARP13, Ago2 and GAPDH (loading control) shown at the right. (d) Bar graphs showing normalized Renilla luminescence for the empty vector and Renilla-TRAILR4 3′UTR, expressed in wild-type (red) or PARP13−/−Acells (blue) treated with control siRNA or siRNA specific for EXOSC5 or XRN1. PARP13-dependent destabilization levels, calculated by substracting normalized Renilla luminescence signal in wild-type cells from the signal in PARP13−/−cells, is shown at the left of the bars. (Means ofn=3 independent replicates, bars show s.d., asterisks represent significance relative to control siRNA destabilization levels, *P<0.05, ***P<0.001,P>0.05 (NS, not significant.) (e) Decay of GAPDH mRNA and TRAILR4 mRNA in wild-type and PARP13−/−cells measured by qRT-PCR of 4-thiouridine incorporated and purified RNA. At each time point GAPDH and TRAILR4 levels were normalized to ACTB levels. Levels at time 0 were set as 0. (Means ofn=3 independent experiments, error bars show s.d., asterisks represent significance relative to wild-type levels for each time point, *P<0.05, **P<0.01, two-sidedt-test.) Figure 6: PARP13 destabilization of TRAILR4 mRNA is exosome dependent. ( a ) TRAILR4 mRNA levels in EXOSC5 and XRN1 knockdowns relative to control knockdown (means of n =3 independent experiments, bars show s.d., asterisks represent significance relative to control siRNA, * P <0.05, P >0.05 (NS, not significant), two-sided t -test). ( b ) Left, EXOSC5 mRNA levels in EXOSC5 knockdown relative to control knockdown (bars show s.d., n =3 independent experiments); right, immunoblot showing XRN1 protein levels in control and XRN1 knockdown. GAPDH is shown as a loading control. ( c ) Relative TRAILR4 mRNA levels in Tet-treated or untreated HEK293 cells expressing Tet-inducible Ago2 shRNA, treated with control or PARP13-specific siRNA (averages of n =3 parallel reactions, error bars show s.d.). Immunoblots of PARP13, Ago2 and GAPDH (loading control) shown at the right. ( d ) Bar graphs showing normalized Renilla luminescence for the empty vector and Renilla-TRAILR4 3′UTR, expressed in wild-type (red) or PARP13 −/−A cells (blue) treated with control siRNA or siRNA specific for EXOSC5 or XRN1. PARP13-dependent destabilization levels, calculated by substracting normalized Renilla luminescence signal in wild-type cells from the signal in PARP13 −/− cells, is shown at the left of the bars. (Means of n =3 independent replicates, bars show s.d., asterisks represent significance relative to control siRNA destabilization levels, * P <0.05, *** P <0.001, P >0.05 (NS, not significant.) ( e ) Decay of GAPDH mRNA and TRAILR4 mRNA in wild-type and PARP13 −/− cells measured by qRT-PCR of 4-thiouridine incorporated and purified RNA. At each time point GAPDH and TRAILR4 levels were normalized to ACTB levels. Levels at time 0 were set as 0. (Means of n =3 independent experiments, error bars show s.d., asterisks represent significance relative to wild-type levels for each time point, * P <0.05, ** P <0.01, two-sided t -test.) Full size image To determine whether exosome or XRN1 activity is required for PARP13-dependent destabilization of TRAILR4 mRNA, we examined the expression of psiCHECK2 reporter constructs encoding Renilla and Renilla-TRAILR4 3′UTR in wild-type and PARP13 −/− cells transfected with control, EXOSC5 or XRN1 siRNA ( Fig. 6d ). Relative PARP13-dependent destabilization was then calculated by subtracting the Renilla/Firefly luciferase signal obtained from wild-type cells from the signal obtained from PARP13 −/− cells ( Fig. 6d ). Knockdown of EXOSC5 resulted in a pronounced defect in the ability of PARP13 to repress TRAILR4 3′UTR with a 15% relative destabilization of the construct compared with 40% in control knockdowns. Knockdown of XRN1 resulted in milder but potentially relevant defects with a 30% relative destabilization of the Renilla-TRAILR4 3′UTR compared with 40% in controls consistent with the observation that exosome activity was the primary pathway regulating endogenous TRAILR4 mRNA ( Fig. 6a ). We therefore conclude that PARP13 requires exosome activity, and potentially XRN1, to destabilize TRAILR4 mRNA (and likely other PARP13 targets). PARP13 decreases TRAILR4 mRNA half-life Since the exosome complex is a key regulator of mRNA decay, we examined the TRAILR4 mRNA decay rate in PARP13 −/− and wild-type cells. Newly transcribed RNA was pulse-labelled with 4-thiouridine and labelled transcripts purified at specific time points after 4-thiouridine removal. qRT-PCR was then performed on the purified transcripts to quantify amounts of TRAILR4 mRNA and GAPDH mRNA. Beta-actin (ACTB) mRNA was used to normalize inputs. TRAILR4 mRNA decay rates were significantly higher in wild-type cells ( t 1/2 =1.5 h) than in PARP13 −/− cells ( t 1/2 =13 h), whereas GAPDH decay rates were similar in both cell lines ( Fig. 6e ). Together, our data are consistent with a model in which PARP13 facilitates efficient degradation of TRAILR4 mRNA via the activity of the exosome complex ( Fig. 6a,d ) and suggest that PARP13 functions as a novel RNA-binding protein that regulates cellular RNA stability by binding to the 3′UTR. PARP13 depletion inhibits TRAIL-induced apoptosis To investigate the physiological relevance of TRAILR4 regulation by PARP13, we examined TRAIL-induced apoptotic signalling upon PARP13 depletion. TRAILR4 expression levels are a key regulator of TRAIL sensitivity in certain cancers [18] , [24] . HeLa cells are TRAIL sensitive due to low TRAILR4 expression, and exogenous expression of TRAILR4 is sufficient to confer TRAIL resistance [21] , [24] ( Fig. 7a ). Of the four TRAIL receptors, only TRAILR4 expression is regulated by PARP13—TRAILR4 mRNA expression, examined by qRT-PCR, and protein levels, assayed by immunoblot, were increased in PARP13 −/− relative to wild-type cells, whereas no differences in protein and mRNA levels of TRAILR1-R2 were identified between PARP13 −/− and wild-type cells, and TRAIL-R3 protein could not be detected in this cell type, consistent with previous reports ( Supplementary Fig. 8 ; Fig. 7b ) [21] . These results suggest that by modulating TRAILR4 expression PARP13 could directly regulate the cellular response to TRAIL. We examined this possibility by assaying TRAIL-induced apoptosis upon PARP13 depletion in TRAIL-sensitive HCT116, SW480 and HeLa cells. Consistent with the increase in TRAILR4 mRNA levels ( Fig. 4d ), PARP13 knockdown resulted in a pronounced resistance to TRAIL treatment in each of these cell types identifying PARP13 as a key regulator of the TRAIL response in these cell lines ( Fig. 7c ). The newly acquired TRAIL resistance was a specific result of increased TRAILR4 expression upon PARP13 knockdown, since simultaneous knockdown of PARP13 and TRAILR4 in HeLa cells resulted in wild-type TRAILR4 mRNA levels and TRAIL sensitivity profiles similar to control knockdowns ( Fig. 7c,d ). 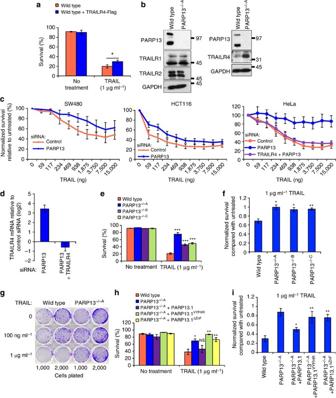Figure 7: PARP13-depletion results in resistance to TRAIL-mediated apoptosis. (a) Percent survival of untreated and TRAIL-treated wild-type cells and wild-type cells expressing TRAILR4-Flag assayed via AnnexinV/propidium iodide (PI) fluorescence-activated cell-sorting (average ofn=3 independent experiments, bars represent s.e.m., *P<0.05, two-sidedt-test). (b) Immunoblot of TRAILR1-2 and TRAILR4 proteins in wild-type and PARP13−/−Acells. GAPDH is used as a loading control. (c) Survival assay measuring proliferation of SW480, HCT116 and HeLa cells with or without PARP13 knockdown after treatment with increasing concentrations of TRAIL for 24 h. Results are shown relative to untreated cells (means ofn=3 independent experiments, error bars show s.e.m.). Results for double knockdown of TRAILR4 and PARP13 are shown for HeLa cells. (d) TRAILR4 mRNA levels after PARP13 and PARP13+TRAILR4 knockdown relative to control knockdown (averages ofn=3 independent experiments, error bars show s.d.). (e) AnnexinV/PI apoptosis assays comparing the percent survival of wild-type and three independent PARP13−/−cell lines (A–C) upon 1 μg ml−1TRAIL treatment for 24 h (n=3 independent experiments, bars show s.e.m., asterisks show significance relative to wild type, ***P<0.001, two-sidedt-test). (f) Normalized survival of wild-type and three PARP13−/−cell lines treated with 1 μg ml−1TRAIL relative to untreated (averages ofn=3 independent experiments, bars show s.e.m., asterisks show significance relative to wild type, *P<0.05 or **P<0.01, two-sidedt-test). (g) Colony-formation assay measured by crystal violet staining of wild-type or PARP13−/−Acells treated with or without the indicated amounts of TRAIL for 7 days. (h) AnnexinV/PI apoptosis assays comparing the percent survival of wild-type, PARP13−/−Aor PARP13−/−Acells expressing PARP13.1, PARP13.1VYFHRor PARP13.1ΔZnFupon treatment with or without 1 μg ml−1TRAIL for 24 h. Data are shown as % survival (means ofn=3 independent experiments, bars show s.e.m., asterisks show significance relative to wild type, *P<0.05, **P<0.01,P>0.05 (NS, not significant), two-sidedt-test). (i) Normalized survival of wild-type, PARP13−/−Acells and PARP13−/−Acells expressing PARP13.1, PARP13.1VYFHRor PARP13.1ΔZnFtreated with 1 μg ml−1TRAIL relative to untreated (n=3 independent experiments, bars show s.e.m., asterisks represent significance relative to wild type, *P<0.05, **P<0.01, ***P<0.001, two-sidedt-test). Figure 7: PARP13-depletion results in resistance to TRAIL-mediated apoptosis. ( a ) Percent survival of untreated and TRAIL-treated wild-type cells and wild-type cells expressing TRAILR4-Flag assayed via AnnexinV/propidium iodide (PI) fluorescence-activated cell-sorting (average of n =3 independent experiments, bars represent s.e.m., * P <0.05, two-sided t -test). ( b ) Immunoblot of TRAILR1-2 and TRAILR4 proteins in wild-type and PARP13 −/−A cells. GAPDH is used as a loading control. ( c ) Survival assay measuring proliferation of SW480, HCT116 and HeLa cells with or without PARP13 knockdown after treatment with increasing concentrations of TRAIL for 24 h. Results are shown relative to untreated cells (means of n =3 independent experiments, error bars show s.e.m.). Results for double knockdown of TRAILR4 and PARP13 are shown for HeLa cells. ( d ) TRAILR4 mRNA levels after PARP13 and PARP13+TRAILR4 knockdown relative to control knockdown (averages of n =3 independent experiments, error bars show s.d.). ( e ) AnnexinV/PI apoptosis assays comparing the percent survival of wild-type and three independent PARP13 −/− cell lines (A–C) upon 1 μg ml −1 TRAIL treatment for 24 h ( n =3 independent experiments, bars show s.e.m., asterisks show significance relative to wild type, *** P <0.001, two-sided t -test). ( f ) Normalized survival of wild-type and three PARP13 −/− cell lines treated with 1 μg ml −1 TRAIL relative to untreated (averages of n =3 independent experiments, bars show s.e.m., asterisks show significance relative to wild type, * P <0.05 or ** P <0.01, two-sided t -test). ( g ) Colony-formation assay measured by crystal violet staining of wild-type or PARP13 −/−A cells treated with or without the indicated amounts of TRAIL for 7 days. ( h ) AnnexinV/PI apoptosis assays comparing the percent survival of wild-type, PARP13 −/−A or PARP13 −/−A cells expressing PARP13.1, PARP13.1 VYFHR or PARP13.1 ΔZnF upon treatment with or without 1 μg ml −1 TRAIL for 24 h. Data are shown as % survival (means of n =3 independent experiments, bars show s.e.m., asterisks show significance relative to wild type, * P <0.05, ** P <0.01, P >0.05 (NS, not significant), two-sided t -test). ( i ) Normalized survival of wild-type, PARP13 −/−A cells and PARP13 −/−A cells expressing PARP13.1, PARP13.1 VYFHR or PARP13.1 ΔZnF treated with 1 μg ml −1 TRAIL relative to untreated ( n =3 independent experiments, bars show s.e.m., asterisks represent significance relative to wild type, * P <0.05, ** P <0.01, *** P <0.001, two-sided t -test). Full size image The TRAIL resistance conferred by PARP13 inhibition can be permanently acquired. PARP13 −/− cells were resistant to both short-term (24 h, Fig. 7e,f ) and long-term TRAIL treatment (7 days, Fig. 7g ), suggesting that one mechanism of TRAIL resistance in cancers could be inhibition of PARP13 function. TRAIL resistance in PARP13 −/− cells was completely reversed by expression of PARP13.1, but not PARP13.1 VYFHR or PARP13.1 ΔZnF , suggesting that the TRAIL resistance in these cells results from the lack of TRAILR4 mRNA regulation by PARP13 ( Fig. 7h,i ). Together these results suggest that PARP13 is necessary and sufficient to regulate the cellular response to TRAIL in cancer cells that are TRAIL sensitive in a manner dependent on TRAILR4 expression. PARP13 depletion abrogates DISC assembly and function TRAILR4 expression levels are important for TRAIL sensitivity in certain cancers due to the receptor’s ability to sequester TRAIL from TRAILR1 and R2 binding, resulting in decreased DISC assembly and apoptotic signalling at these receptors upon TRAIL treatment. This apoptotic signalling is mediated by caspase-8, which is recruited to the DISC where it is activated and autoprocesses itself. Thus caspase-8 cleavage can be used to directly report on caspase-8 enzymatic activity. To determine whether the TRAIL resistance observed in PARP13 −/− cells results from attenuated apoptotic signalling at the TRAIL receptor level, time-dependent caspase-8 processing was analysed in wild-type or PARP13 −/−A cells treated with TRAIL. Whereas caspase-8 was processed in HeLa cells resulting in the appearance of p43/p41 and p18 fragments, no such processing was observed in PARP13 −/− cells, demonstrating an ablation of DISC signalling ( Fig. 8a ). A consistent upregulation of both PARP13.1 and PARP13.2 was observed upon TRAIL treatment suggesting positive feedback signalling ( Fig. 8a ). To determine whether DISC assembly itself is defective in PARP13 −/− cells, we compared assembly with wild-type cells using standard DISC precipitation assays that utilize epitope-tagged TRAIL [36] . Recruitment of TRAILR1, TRAILR2 and caspase-8 to the DISC was greatly diminished in PARP13 −/− cells relative to wild type ( Fig. 8b ). Together these results suggest that the TRAIL resistance found upon PARP13 depletion is due to defective DISC assembly, decreased caspase-8 activation and decreased apoptotic signalling from TRAIL receptors. 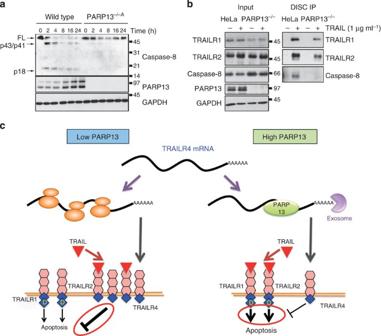Figure 8: PARP13 depletion inhibits the formation of a functional DISC complex. (a) Immunoblot examining caspase-8 cleavage at various time points after 1 μg ml−1TRAIL treatment in wild-type and PARP13−/−cells. Arrows indicate full-length (FL) caspase-8 and its cleavage products. GAPDH shown as a loading control. (b) Flag-TRAIL pulldown of the TRAIL–receptor complex in wild-type and PARP13−/−Acells blotted for TRAILR1, R2 and caspase-8. Inputs for the reaction are also shown. (c) Model of PARP13-dependent TRAILR4 mRNA regulation and its effects on TRAIL-mediated apoptosis. Figure 8: PARP13 depletion inhibits the formation of a functional DISC complex. ( a ) Immunoblot examining caspase-8 cleavage at various time points after 1 μg ml −1 TRAIL treatment in wild-type and PARP13 −/− cells. Arrows indicate full-length (FL) caspase-8 and its cleavage products. GAPDH shown as a loading control. ( b ) Flag-TRAIL pulldown of the TRAIL–receptor complex in wild-type and PARP13 −/−A cells blotted for TRAILR1, R2 and caspase-8. Inputs for the reaction are also shown. ( c ) Model of PARP13-dependent TRAILR4 mRNA regulation and its effects on TRAIL-mediated apoptosis. Full size image In this manuscript we show that PARP13 binds cellular RNA and that its depletion results in significant misregulation of the transcriptome with an enrichment in signal peptide-containing transcripts and immune response genes. We identify the mRNA encoding TRAILR4 as the first experimentally verified cellular target of PARP13 repression, and demonstrate that PARP13 destabilizes TRAILR4 mRNA post-transcriptionally by binding to its 3′UTR and targeting it for degradation via the exosome complex. Consistent with these data, PARP13 depletion markedly alters TRAILR4 mRNA decay kinetics. By repressing TRAILR4 expression in the cell, PARP13 shifts the balance in the TRAIL signalling pathway towards decreased anti-apoptotic signalling and sensitizes cells to TRAIL-mediated apoptosis ( Fig. 8c ). Expression of decoy receptors has been described as one mechanism of TRAIL resistance in cancer [17] , [36] . Our results suggest that PARP13 could have important functions in regulating TRAIL resistance and that modulation of PARP13 may have the potential to overcome TRAILR4-mediated TRAIL resistance. This approach could improve the efficacy of TRAIL therapies currently in clinical trials to target multiple cancers [37] . Furthermore, it was recently shown that PARP1/2 inhibitors result in transcriptional upregulation of TRAILR2 and subsequent apoptosis in acute myeloid leukaemias [38] . It therefore appears that the cellular response to TRAIL is regulated by multiple PARPs via transcriptional and post-transcriptional mechanisms. Several important questions remain regarding PARP13 function in the regulation of cellular mRNA—what are the direct targets of regulation, how is target specificity determined and does the regulation of cellular targets change upon viral infection? With the exception of TRAILR4, many of the transcripts misregulated upon PARP13 knockdown identified in this work are likely indirect targets. To better understand the biology of PARP13, identifying additional direct targets will be critical. On the basis of previous research on the selectivity of viral RNA binding to PARP13, target recognition of cellular mRNA is more likely to be mediated by structural features rather than linear sequence motifs, therefore it is unlikely that a consensus sequence will be identified [6] , [13] . Interestingly, the expanded ARE in the TRAILR4 3′UTR is predicted to form a hairpin with high probability ( Supplementary Fig. 5 ), suggesting that it may represent a structure recognized by PARP13 (ref. 34 ). The highly significant enrichment of signal peptide-containing transcripts upon PARP13 depletion (corrected P value <0.0001) strongly suggests that PARP13 has a specific function in the regulation of transmembrane proteins, or those that are destined to be secreted. This enrichment might be related to PARP13.1 localization at the ER. Indeed, PARP13.1 has been shown to be farnesylated, and this modification targets PARP13.1 to membranes and is required for its antiviral activity [2] . It is therefore possible that similar targeting of PARP13.1 to membranes might also regulate its function in destabilizing cellular transcripts, including those at the ER. It is important to note that PARP13 is just one member of the CCCH PARP subfamily identified based on the presence of CCCH zinc finger RNA-binding domains—PARP12 and PARP7 are the other two members [1] . Whereas PARP7 is poorly studied and little is known about its function, both PARP12 and PARP13 function in the antiviral response and localize to membraneous organelles (PARP13 to the ER and PARP12 to the Golgi) [1] , [39] , [40] . In addition, PARP12 and PARP13 exhibit similar domain structures including the presence of multiple tandem CCCH zinc-fingers (vs only one in PARP7) [1] . Therefore PARP12 might also regulate cellular RNA in a manner similar to PARP13. General Experiments were performed in HeLa Kyoto cells unless otherwise stated. Knockdowns were performed using Lipofectamine 2000 as per the manufacturer’s instructions with double transfections of 48 h. Exogenously expressed constructs were transfected using Lipofectamine 2000 for 24 h before the assay. Mutants were cloned using GeneString technology. TRAILR4 3′UTR was cloned from Origene clone SC117708 into psiCHECK2 using GeneString technology. TRAILR4 3′UTR fragments were cloned by PCR amplification of the indicated regions and cloned into psiCHECK2. Renilla and Firefly luminescence were measured 48 h post transfection. Crosslinking followed by immunoprecipitation was performed as previously described [41] . To assess cell sensitivity to TRAIL-mediated apoptosis, cells were treated with TRAIL for 24 h, and cell viability was assayed by the MTT assay (Millipore) or by Annexin V/PI flow cytometry (Biolegend) as per the manufacturer’s instructions. Standard western blotting techniques were used, and full scans of important blots along with protein ladder markers are shown in Supplementary Fig. 9 . Cell culture and transfection Cells were grown at 37 °C and 5% CO 2 . HeLa Kyoto (ATCC), SW480 (a gift from Ryoma Ohi, Vanderbilt) and HEK293 (ATCC) cells were maintained in Dulbecco's modified Eagle's medium (DMEM) (Invitrogen) supplemented with 10% fetal bovine serum (Life Technologies); hTERT-RPE1 cells (ATCC) in Ham’s F12/DMEM (Mediatech) supplemented with 10% fetal bovine serum and HCT116 cells (ATCC) were cultured in McCoy’s 5A (ATCC) supplemented with 10% fetal bovine serum (Life Technologies). For expression of recombinant proteins, HeLa cells were transfected with Lipofectamine 2000 (Life Technologies) 24 h prior to the assay. For RNA interference, two 48-h transfections were performed with 20 nM siRNA for Stealth siRNAs or 5 nM for Silencer Select siRNAs using Lipofectamine 2000 according to the manufacturer’s protocol. For RPE1 RNA interference, 5 nM of siRNA was transfected with Silentfect (Bio-Rad) following the manufacturer’s protocols. IFNγ was from R&D Serotec, JAKi from Calbiochem and Flag-TRAIL from Axxora. His-TRAIL was purified according to standard procedures [42] . PARP13 knockout cell lines Zinc-finger nucleases specific to the PARP13 genomic locus were purchased from Sigma Aldrich and transfected into HeLa Kyoto cells. Monoclonal cell lines (PARP13 −/− A/B/C) were generated using serial dilution in 96-well plates, then tested for PARP13 expression via western blot. Three independent monoclonal cell lines lacking PARP13 expression were generated. Cloning Green fluorescent protein (GFP)-PARP13 has been described previously [1] . To generate SBP-PARP13, GFP was substituted with the streptavidin-binding peptide tag using NheI and BspEI. PARP13 ΔZnF and PARP13 RNA-binding point mutants were generated using GeneString (Invitrogen) flanked by XhoI/BstXI, which are internal sites in PARP13. PARP13 ΔZnF features a deletion from nt228 to nt669. The psiCHECK2 vector encoding Renilla and Firefly luciferase genes was purchased from Promega. TRAILR4 ORF was purchased from Origene (SC117708). A SalI site was introduced after the TRAILR4 stop codon using a Gene String flanked by PpuMI and ScaI, which are internal sites in TRAILR4 complementary DNA (cDNA). The 3′UTR of TRAILR4 was then introduced downstream the Renilla luciferase in psiCHECK2 using SalI/XhoI and NotI digestion. psiCHECK2+GAPDH 3′UTR is a kind gift from Dr Benilde Jimenez. Truncations of TRAILR4 3′UTR were generated by PCR using primers with XhoI/NotI overhangs. psiCHECK2+TRAILR4 3′UTR was used as a template. Fragments were designed based on TRAILR4 3′UTR folding prediction (RNAFold) so as to preserve high-probability folding structures [34] . Total RNA purification and Agilent microarrays Total RNA purification was performed using the Qiagen RNeasy Kit following the manufacturer’s instructions. Samples were labelled using the Two Color Quick Amp Labeling Kit (Agilent) following the manufacturer’s protocol and hybridized on SurePrint G3 Human Gene Expression v2 8 × 60 microarray. Microarrays were scanned on the SureScan Microarray Scanner (Agilent) and processed with Feature Extractor v10.5. Microarrays have been submitted to GEO, NCBI; accession number GSE56667 . CLIP HeLa cells were ultraviolet-crosslinked at 254 nm with 200 mJ cm −2 (Stratagene Stratalinker). For endogenous PARP13 immunoprecipitation, cells were lysed in CLIP lysis buffer (1% NP-40, 0.1% SDS, 150 mM NaCl, 1 mM EDTA, 50 mM TRIS (pH 7.4) and 1 mM dithiothreitol (DTT)), precleared at 16,100 g , treated with RNaseA for 10 min at 37° C, immunoprecipitated overnight with PARP13 antibody and washed 2 × in CLIP lysis buffer containing 1 M NaCl. Bound RNA was labelled and detected according to Leung et al . [41] For SBP-PARP13 precipitation, cells were ultraviolet-crosslinked as described above, lysed with cell lysis buffer (CLB) (150 mM NaCl, 50 mM HEPES (pH 7.4), 1 mM MgCl 2 , 0.5% Triton, 1 mM EGTA and 1 mM DTT), precleared at 16,100 g , incubated with RNase A for 10 min at 37° C and bound to Streptavidin Sepharose beads (GE Healthcare). RNA bound to SBP-PARP13 was labelled according to Leung et al . [41] and bound protein eluted with 4 mM biotin. CLIP qRT-PCR Cells were ultraviolet-crosslinked at 254 nM 200 mV cm −2 and lysed in 1% Triton, 125 mM KCl, 1 mM EDTA and 20 mM HEPES pH 7.9 under RNase-free conditions. SBP-PARP13 and PARP13 mutants were immunoprecipitated using Streptavidin Sepharose beads. After binding, beads were washed with lysis buffer supplemented with 10 μg ml −1 tRNA and 250 mM KCl. Proteins were eluted in 4 mM biotin, treated with proteinase K and RNA was purified using Trizol, following the manufacturer’s protocol. Input RNA was collected similarly from total lysate before the immunoprecipitation step. cDNA was prepared from input and bound RNA as described below. qRT-PCR cDNA was prepared using the ViLo First Strand Kit (Life Technologies) and random primers. 1 μg of total RNA or all CLIP-bound RNA was used per reaction. 100 ng cDNA was used for each qRT-PCR reaction. Sybr Select reagent (Life Technologies) was used as directed and qRT-PCR was performed on a Roche 480 Light Cycler. Data analysis was performed as previously described [43] , using the ΔΔcT method. In all cases ACTB was used as a normalizing control. For gene-specific qRT-PCR primers used in this manuscript refer to Supplementary Table 1 . Dual luciferase assays HeLa cells were transfected with 50 ng of psiCHECK2 constructs in 24-well plates. Forty-eight-hour post-transfection cells were lysed and lysates treated with the Pierce Renilla-Firefly Dual Luciferase Assay Kit as per instructions (Thermo Scientific). Firefly and Renilla luminescence was measured in white 96-well plates in a Tecan Plate Reader (Magenta and Green, 1,000 ms each). Renilla luminescence signal was normalized to the Firefly signal for each well. For all figures bars represent averages of three individual 24-well plate wells; error bars represent s.d. Cell staining and microscopy Cells were split onto glass coverslips 16 h before treatment. To induce cytoplasmic stress, cells were incubated with 200 μM sodium arsenite for 45 min at 37° C; control cells were left untreated. Unstressed cells were fixed in 4% formaldehyde for 30 min then extracted with Abdil 0.5% Triton for 25 min. Stressed cells were pre-extracted with HEPES buffered saline buffer (HBS) containing 0.1% Triton for 1 min, then fixed in 4% formaldehyde in HBS for 30 min. Blocking and staining was performed as previously described [1] . Fixed cells were blocked in Abdil (4% bovine serum albumin (BSA), 0.1% Triton in phosphate-buffered saline (PBS)), then incubated with antibodies diluted in Abdil for 45 min each. Survival assay For proliferation assays, 5,000 cells were plated in 96-well plates and incubated with recombinant TRAIL the following day for 24 h. Proliferation was analysed with the Cell Proliferation Kit II (Roche) according to the manufacturer’s instructions and survival was calculated by normalizing treated to untreated cells. For apoptosis assays, 40,000 cells were plated in 24-well plates and incubated with recombinant TRAIL for 24 h. Cells were harvested with trypsin and stained with Annexin V-488 (Biolegend) and propidium iodide (Sigma) in Annexin binding buffer (10 mM HEPES, 140 mM NaCl and 2.5 mM CaCl 2 , pH 7.4) for 15 min at room temperature. Fluorescence-activated cell-sorting analysis was performed on a FACScan instrument (BD) and cells negative for Annexin V and propidium iodide were considered as alive. For colony-forming assays, the indicated numbers of cells were plated in 12-well plates and grown for 7 days in medium with TRAIL changed every second day. Colonies were visualized by staining with 0.02% crystal violet (Sigma) in 50% methanol. Electrophoretic mobility shift assays SBP-PARP13.1 and SBP-PARP13.1 VYFHR were purified from HEK293 cells lysed with CLB (150 mM NaCl, 50 mM HEPES (pH 7.4), 1 mM MgCl 2 , 0.5% Triton, 1 mM EGTA and 1 mM DTT), precleared at 80,000 g and bound to Streptavidin Sepharose beads (GE Healthcare). Beads were washed with CLB containing 1 M NaCl, and proteins were eluted with 4 mM biotin in CLB, then dialysed overnight in 100 mM KCl, 50 mM TRIS, pH 7.5. Protein concentrations were determined by Coomassie blue stain by comparison with a dilution series of BSA, and by ultraviolet spectrophotometry. Fragment 1 and fragment E were PCR-amplified, in vitro transcribed using T7 RNA polymerase, purified and end-labelled with T4 polynucleotide kinase and 32 P γATP as previously described [44] . EMSA-binding reactions were performed for 1 h at 20° C in 10 mM Tris, pH 7.5, 1 mM EDTA, pH 8, 0.1 M KCl, 0.1 mM DTT, 5% vol/vol glycerol, 0.01 mg ml −1 BSA, 0.4 units μl −1 RNAse inhibitor, 0.1 μg ml −1 tRNA with 2 nM RNA and decreasing amounts of protein. Reactions were loaded onto 8% Tris/borate/EDTA buffer (TBE) urea gels, and run in 0.5 × TBE at room temperature, then exposed to phosphor screen and scanned. To calculate Kd, bands were quantified using ImageJ, fraction bound was calculated, and data were fit to Hill’s equation using IGOR Pro. 4-thiouridine labelling and mRNA decay measurements Wild-type and PARP13 −/−A cells were incubated with 200 μM 4-thioruridine for 2 h, then growth media was changed and cells were collected immediately, and at 2-h intervals for 8 h. Total RNA was Trizol extracted at each time point and newly transcribed RNA was biotin-labelled and purified as previously described [45] . In brief, newly transcribed RNA was labelled with biotin-HPDP (N-[6-(biotinamido)hexyl]-3′-(2′-pyridyldithio)propionamide), RNA was repurified and newly transcribed RNA was separated on streptavidin-coated magnetic beads (Miltenyi). RNA was eluted with 100 mM DTT, and purified using the MinElute Cleanup Kit (Qiagen). RT-qPCR was performed as described above. TRAILR4 and GAPDH levels were normalized to ACTB for each sample. Each time point represents an average of three independent experiments; error bars show the s.d. Half-life was calculated as previously described [46] . Half-life is an underestimate as expression levels are normalized to ACTB levels, which are also decreasing within this time course (ACTB half-life in HeLa cells is ~8 h (ref. 47 )). DISC-IP Wild-type or Parp13 −/−A cells (1 × 10 6 ) each were plated in two 10-cm plates for 2 days. Plates were washed once in DMEM (without fetal calf serum) and then incubated for 45 min in 2.5 ml DMEM without fetal calf serum and with or without 1 μg ml −1 Flag-TRAIL (Axxora). After addition of 15 ml cold PBS, cells were washed once with 15 ml cold PBS and scraped with a rubber policeman in 1 ml lysis buffer (30 mM Tris/HCl pH 7.4, 150 mM NaCl, 5 mM KCl, 10% glycerol, 2 mM EDTA and protease inhibitors). After addition of 100 μl Triton X-100, lysates were rotated 30 min at 4 °C and harvested by centrifugation (45 min, 4 °C, 15,000 g ). The supernatant was removed, added to 20 μl magnetic Protein-G beads (Invitrogen), washed three times in lysis buffer including Triton X-100 and rotated at 4° C overnight. After five washes in lysis buffer including Triton X-100, beads were heated at 75° C for 10 min in 20 μl loading buffer, subsequently loaded on a gel and blotted for the indicated antibodies. Caspase-8 processing Wild-type and PARP13 −/− cells were plated in six wells and treated with His-TRAIL for the indicated time periods. Cells were harvested, lysed and analysed by immunoblot with the indicated antibodies. Reagents used in this manuscript For reagents used please refer to Supplementary Table 1 . How to cite this article: Todorova, T. et al . PARP13 regulates cellular mRNA post-transcriptionally and functions as a pro-apoptotic factor by destabilizing TRAILR4 transcript. Nat. Commun. 5:5362 doi: 10.1038/ncomms6362 (2014). Acccssion codes: Microarray data for control and PARP13 knockdowns have been submitted to the NCBI Gene Expression Omnibus under accession code GSE56667.